Silicon nanofin grating as a miniature chirality-distinguishing beam-splitter The polarization of light plays a central role in its interaction with matter, in situations ranging from familiar (for example, reflection and transmission at an interface) to sophisticated (for example, nonlinear optics). Polarization control is therefore pivotal for many optical systems, and achieved using bulk devices such as wave-plates and beam-splitters. The move towards optical system miniaturization therefore motivates the development of micro- and nanostructures for polarization control. For such control to be complete, one must distinguish not only between linear polarizations, but also between left- and right-circular polarizations. Some previous works used surface plasmons to this end, but these are inherently lossy. Other works used complex-layered structures. Here we demonstrate a planar dielectric chirality-distinguishing beam-splitter. The beam-splitter consists of amorphous silicon nanofins on a glass substrate and deflects left- and right-circularly polarized beams into different directions. Contrary to intuitive expectations, we utilize an achiral architecture to realize a chiral beam-splitting functionality. Along with its wavelength and propagation direction, the polarization of light is one of its basic attributes. Light–matter interactions, from simple Fresnel reflections [1] to single-molecule spectroscopy [2] , can be highly polarization dependent. It is for this reason that polarization control is essential for major classes of optical systems such as free-space, fibre-optic and on-chip systems. In some free-space optical systems, such as compact disc and digital versatile disc players, polarization control enables the separation of incident and reflected beams with high efficiency [3] . Others, such as ellipsometers [4] and imaging systems [5] , aim to characterize materials and scenes via their response to polarized light. The benefits of polarization-resolved imaging are evidenced by the fact that some animal eyes have evolved to achieve this functionality, for example, the mantis shrimp can resolve the full polarization state of light (Stokes vectors) [6] . Indeed, polarization-resolved imaging can enhance contrast [7] , [8] and enable the classification of chemical isomers [9] . In both fibre-optic [10] and on-chip [11] systems, polarization control is needed to prevent the detrimental effects of polarization-mode dispersion. We also note that, in addition to its importance in optical system design, it has been predicted that polarization control in metamaterials can provide unusual properties such as negative refraction [12] . The continuous trend towards miniaturization has generated considerable interest in polarization control devices based on micro- and nanostructures. It has been known for some time [13] that wire-grids act as linear polarizers [14] , and recent work has demonstrated their integration with image sensor devices for division-of-focal-plane-imaging polarimeters [5] . For full control over polarization, however, the ability to distinguish between left- and right-circularly polarized (LCP, RCP) light is crucial. This has led to intense interest in the development of plasmonic and photonic nanostructures that achieve this aim. Thus far, these have largely comprised devices with circular dichroism and optical activity [15] , [16] , [17] , [18] , [19] , [20] , [21] , [22] , [23] . The former refers to differences in absorption between LCP and RCP. The latter refers to the rotation of the plane of polarized light upon passing through the device. There has also been interest in nanostructures that produce superchiral fields [24] , due to the fact that many molecules important in biology and chemistry are chiral and respond very differently to LCP and RCP light [25] . Largely, however, the nanostructures developed thus far that distinguish between LCP and RCP can be thought of as filters and wave-plates. An ubiquitous functionality employed in systems based on bulk optics, however, is that of beam-splitting. This motivates the development of chiral beam-splitters that separate LCP from RCP. Turner et al. [26] recently demonstrated a chiral beam-splitter based on a gyroid photonic crystal. The device was fabricated by direct laser writing and comprised a triangular prism with an overall size of 96 × 96 × 24 μm 3 , or 64,000 cubic unit cells ( a =1.2 μm). For many applications, however, achieving the chiral beam-splitting functionality using a single nanostructured layer fabricated by one conventional lithography step, rather than a bulk photonic crystal fabricated by three-dimensional (3D) direct laser writing [26] , would be preferable. Here, we demonstrate a planar chirality-distinguishing beam-splitter (CDBS) consisting of amorphous silicon (a-Si) nanofins on a glass substrate. We show by simulation and experiment that our structure deflects LCP and RCP beams into different directions. Interestingly, our approach is conceptually different from previous methods for distinguishing LCP from RCP that made use of chiral structures, for example, see refs 15 , 16 , 17 , 18 , 19 , 20 , 21 , 22 , 23 . By contrast, our device is achiral and possesses neither intrinsic [15] , [16] , [17] , [18] , [19] , [20] , [21] , [22] , [23] nor extrinsic [27] , [28] chirality (see Supplementary Fig. 1 and Note 1 ). The mechanism by which it distinguishes between LCP and RCP is discussed in the following section. Silicon nanofins as birefringent media A schematic diagram of our CDBS device is shown in Fig. 1a . The device comprises unit cells ( Fig. 1b,c ) that are each 3 μm × 0.5 μm ( P x =3 μm, P y =0.5 μm). Each unit cell contains six nanofins that successively rotate by θ =30° and are spaced by 0.5 μm, centre-to-centre. The guideline we adopted for device design is discussed in the Supplementary Note 2 . Similar to other nanostructures with azimuthal asymmetry, nanofins exhibit form birefringence [29] . This can be understood by considering that a single nanofin resembles a channel waveguide. An optical mode whose electric field is polarized along the nanofin long axis (here denoted as extraordinary axis, or e axis, Fig. 1d ) will have a larger effective mode index than the one polarized along the short axis (here denoted as ordinary axis, or o axis). To quantify this effect, we perform electromagnetic simulations to find the effective mode indices ( n e and n o ) along the e - and o -axes as a function of nanofin width W (dimension along the o axis, Fig. 1d ), with the nanofin length L (dimension along the e axis) maintained at 300 nm. These are performed using the beam propagation method (BPM) for a single (isolated) a-Si nanofin suspended in air. The simulation results ( Fig. 2a ) demonstrate that significantly different effective indices are obtained depending on the input polarization. Also shown in the same figure is the phase retardation between the two polarizations for a propagation length of 1 μm. A phase retardation as large as 2 π can be achieved, confirming the role of the nanofin as a wave-plate. To further illustrate this effect for periodic arrays of nanofins, we performed simulations using the finite difference time domain (FDTD) method. Each nanofin has a width W =50 nm and length L =300 nm. The nanofins are arranged in a square lattice with a spacing of 0.5 μm and they are on a glass substrate. A unit cell of the simulated structure is shown in Fig. 1f . Periodic boundary conditions are applied at the x - and y -boundaries, and perfectly matched layers (PMLs) are applied at the z -boundaries. The use of the PML at the + z -boundary (to which the nanofin extends) results in an infinitely long nanofin being modelled. This eliminates the reflection and scattering that would otherwise occur at the end of the nanofin and the resultant Fabry–Perot interference that would complicate the analysis. Instantaneous field distributions are shown in Fig. 2b,c . Figure 2b presents the x -component of the electric field, with the input illumination (from substrate) also x -polarized. 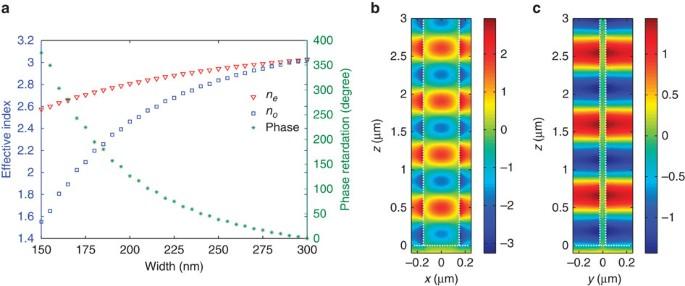Figure 2: Birefringence effects in silicon nanofins. (a) Effective mode index of single (isolated) nanofin versus its width, when excited either along the nanofineaxis (ne) oroaxis (no). For these simulations, the nanofin is assumed to be suspended in the air and has a lengthL=300 nm. Phase retardation between these two electric field components is also shown for a propagation length of 1 μm. (b) Instantaneous electric field (x-component) distribution of nanofin inx–zplane for the case ofx-polarized plane-wave illumination. (c) Instantaneous electric field (y-component) distribution of nanofin iny–zplane for the case ofy-polarized plane-wave illumination. All simulations are performed at a wavelength of 975 nm. Similarly, Fig. 2c presents the y -component of the electric field, with the input illumination (from substrate) also y -polarized. It can be seen that the nanofin supports guided modes with flat phase fronts (see Supplementary Fig. 2 and Note 3 ). This flat phase confirms presence of a dominant guided mode, and the absence of radiation modes, resulting in minimal scattering loss. The results show a prominent difference between the modes, depending on whether the electric field is along the e axis or o axis ( Fig. 2b,c ), confirming the birefringent nature of the nanofins in a two-dimensional periodic array. Although our nanofin grating ( Fig. 1a ) is achiral, we employ the nanofin birefringence to achieve a CDBS functionality. 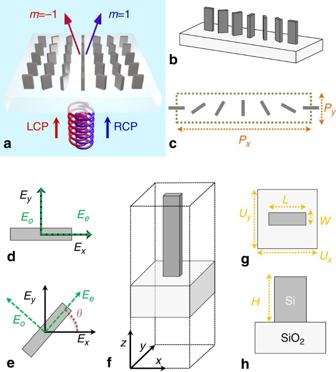We further describe the operating principle next. Figure 1: Schematic diagram of a chirality-distinguishing beam-splitter (CDBS). (a) CDBS device consists of a-Si nanofin grating on a glass substrate, and redirects the impinging light based on its handedness. (b,c) Side- and top-views of unit cell of nanofin grating. Unit cell contains six nanofins, spaced by 500 nm (centre-to-centre) that successively rotate. (d) Cross-section of single nanofin in which crystal (nanofin) coordinates (e- andoaxes) coincides with laboratory coordinates (x- andyaxes). (e) Rotation of nanofin by angleθresults in a mismatch between crystal and laboratory coordinates. (f) Schematic diagram of a-Si nanofin on a glass substrate. Periodic boundary conditions are applied atx-andy-boundaries, and perfectly matched layers (PMLs) atz-boundaries. (g) Top-view of a nanofin, showing widthW, lengthLand size of the unit cell (Ux=Uy=500 nm). (h) Side-view of a nanofin, showing heightH. Plane of incidence and propagation direction of incident beam arex–zand+z, respectively. Figure 1: Schematic diagram of a chirality-distinguishing beam-splitter (CDBS). ( a ) CDBS device consists of a-Si nanofin grating on a glass substrate, and redirects the impinging light based on its handedness. ( b , c ) Side- and top-views of unit cell of nanofin grating. Unit cell contains six nanofins, spaced by 500 nm (centre-to-centre) that successively rotate. ( d ) Cross-section of single nanofin in which crystal (nanofin) coordinates ( e - and o axes) coincides with laboratory coordinates ( x - and y axes). ( e ) Rotation of nanofin by angle θ results in a mismatch between crystal and laboratory coordinates. ( f ) Schematic diagram of a-Si nanofin on a glass substrate. Periodic boundary conditions are applied at x- and y- boundaries, and perfectly matched layers (PMLs) at z -boundaries. ( g ) Top-view of a nanofin, showing width W , length L and size of the unit cell ( U x = U y =500 nm). ( h ) Side-view of a nanofin, showing height H . Plane of incidence and propagation direction of incident beam are x–z and +z , respectively. Full size image Figure 2: Birefringence effects in silicon nanofins. ( a ) Effective mode index of single (isolated) nanofin versus its width, when excited either along the nanofin e axis ( n e ) or o axis ( n o ). For these simulations, the nanofin is assumed to be suspended in the air and has a length L =300 nm. Phase retardation between these two electric field components is also shown for a propagation length of 1 μm. ( b ) Instantaneous electric field ( x -component) distribution of nanofin in x – z plane for the case of x -polarized plane-wave illumination. ( c ) Instantaneous electric field ( y -component) distribution of nanofin in y – z plane for the case of y -polarized plane-wave illumination. All simulations are performed at a wavelength of 975 nm. Full size image Operating principle As discussed above, birefringence originates from the asymmetric cross-section ( L > W) of the nanofin. Each nanofin thus acts like a wave-plate and its transmission can be modelled by Jones matrix, here denoted J ( θ , ϕ ). To find this matrix, we need to take into account its orientation ( θ ) with respect to the laboratory coordinate frame ( x and y axes, Fig. 1e ). The Jones matrix of a wave-plate [30] is given by the product of the matrix R(θ) that transforms from the laboratory to crystal (here: nanofin) coordinate frames, the Jones matrix in crystal coordinates J 0 and the matrix R(−θ) that transforms back to the laboratory coordinate frame: The quantity ϕ represents the phase retardation between the propagating extraordinary and ordinary components, which are polarized parallel to the length ( e axis) and width ( o axis) of the nanofin, respectively ( Fig. 1d ). We now use this to predict the far-field response of our nanofin grating. This comprises diffracted orders whose electric fields are the vectorial Fourier components of the transmitted field [31] : E out ( m ) is a vector that gives the electric field of the m -th diffracted order. Its first entry gives the electric field polarized along the direction perpendicular to the propagation direction and the y axis. Its second entry gives the electric field polarized along the y axis. E in is a vector denoting the input electric field, and its entries give the electric fields polarized along the x - and y axes. We note that as the device has sub-wavelength periodicity along the y axis and is under normal incidence excitation, the integration only needs to be performed along the x axis. Equation (2) implies that, as θ is a function of x , one can tailor the electric field distribution in the near-field and thus control the output electric field in the far-field. This can be done by appropriate design of the grating unit cell. Here, we use this approach to realize a CDBS. We consider array of unit cells, each of which consists of a-Si nanofins that successively rotate as one moves along the x -direction ( Fig. 1a,c ). θ is therefore a function of x as θ = πx / P x , with the assumption that the discrete nature of the device (that is, there are six nanofins per unit cell) can be ignored. This assumption is advantageous for physical interpretation. We will furthermore see later that the prediction of the CDBS functionality that results from this assumption is confirmed by FDTD simulations of the actual structure (that is, that include its discrete nature). Substituting θ in equation (2) shows that there are only three possible diffracted orders ( m =0, ±1): This result is derived in Supplementary Note 4 . It can be seen that the power in the m =0 diffracted order does not depend on the phase difference between incident electric field components. On the other hand, the powers of the m =±1 orders are sensitive to the phase difference. This characteristic enables us to identify the handedness of the incident light through observation of the m =±1 orders. Furthermore, the fraction of power that is in the m =±1 orders versus the m =0 order can be varied from zero to 100% by appropriate choice of phase retardation ϕ . The latter can be achieved by adjusting the nanofin dimensions or changing the surrounding refractive index (see Supplementary Fig. 3 and Note 5 ). If ϕ is an odd multiple of π , the output is entirely first order ( m =±1), while if ϕ is an even multiple of π , the output is entirely zero-th order ( m =0). Device fabrication and far-field measurements Scanning electron micrographs show top-view ( Fig. 3a ) and side-view ( Fig. 3b ) images of the fabricated a-Si nanofin grating. The unit cell is denoted by a dashed red rectangle in the top-view scanning electron micrograph of Fig. 3a . 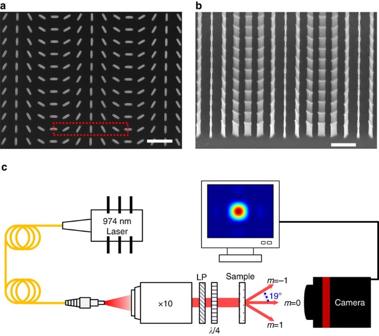Figure 3: Fabricated device and measurement setup. (a) Top-view scanning electron micrograph (SEM) of a fabricated chirality-distinguishing beam-splitter (CDBS) device (a-Si nanofin grating). Dashed red rectangle indicates unit cell. Scale bar, 1 μm. (b) Side-view SEM of a CDBS device. Nanofins are slightly tapered in the minor axis, whereas tapering in the major axis is negligible. Aluminium mask is visible in this SEM, but removed before optical measurements. Scale bar, 1 μm. (c) Experimental setup consists of a fiber-coupled laser (λ=974 nm) whose beam is collimated and passes through a linear polarizer (LP: maintained at 45°) and a quarter-wave-plate (λ/4) to generate the desired input polarization. Angle between zero-th and first order is measured to be 19°. Figure 3c shows the experimental setup used to characterize the device. We measure the far-field intensities of the zero-th and first orders under linearly polarized ( Fig. 4a,c ), LCP ( Fig. 4d–f ) and RCP ( Fig. 4g–i ) illumination. The nanofins have top widths ( W ), lengths ( L ) and heights ( H ) of 55, 285 and 1,500 nm, respectively. The a-Si deposition thickness is 1,680 nm, and there is thus a residual layer (180 nm thick) of a-Si. The nanofins are also slightly tapered, with a base width of 85 nm. The transmitted light is either captured by a camera or collected by a photodetector (power meter). 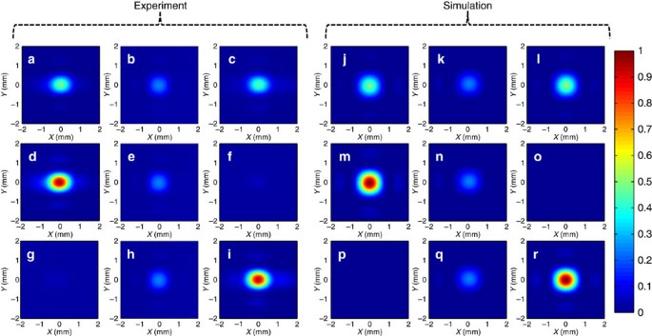Figure 4: Comparison between measurements and simulations. Measured intensities of (a) −1 order (b) zero order and (c) +1 order for linearly polarized illumination. Measured intensities of (d) −1 order (e) zero order and (f) +1 order for left-circularly polarized (LCP) illumination. Measured intensities of (g) −1 order (h) zero order and (i) +1 order for right-circularly polarized (RCP) illumination. Corresponding simulations for linearly polarized (j–l), LCP (m–o) and RCP (p–r) illumination. Simulations are performed for nanofins with top widths of 55 nm, base widths of 70 nm, lengths of 285 nm and heights of 1,500 nm. These dimensions are chosen to match those found from scanning electron micrographs of a fabricated chirality-distinguishing beam-splitter device, but with base width modified. Figure 4a–c show the measured m =−1, m= 0 and m =+1 orders, respectively, as captured by the camera for linearly polarized illumination. We measure the angle of the first order to be at φ =19° from the normal to the substrate. This angle agrees with expectations ( φ =sin −1 ( λ / P x )≈19°). In addition, the diffraction angle can be tuned by modifying the value of P x . This can be achieved by changing the spacing between neighbouring nanofins along the x axis or by maintaining their spacing and changing the number of nanofins in each unit cell (and modifying the rotation angle θ accordingly). This is shown in Supplementary Figs 4 and 5 and Note 6 . For linearly polarized illumination, we measure the powers of the m =−1, m =0 and m =+1 orders as being 38, 20 and 38% of transmitted power, respectively. In addition, the second orders ( m =±2) receive 4% of the transmitted power. On the basis of theory and simulation we should not have second orders, but their presence is inevitable in the actual device due to imperfection in fabrication. The experimental results are in good agreement with simulations ( Fig. 4j–l ) that predict values of 40, 20 and 40% for the m =−1, m =0 and m =+1 orders, respectively. These simulations are performed using the FDTD method for nanofins with dimensions matching those of fabricated devices, except with the base width modified to be 70 nm. It is found that this modification results in an improved fit to the experimental results. We next demonstrate that our device is indeed a CDBS. For LCP illumination ( Fig. 4d–f ), as expected, the measured zero-th order’s power does not change, but the m =−1 order increases to ~76% while the m =+1 order approaches zero. This trend is in agreement with simulations ( Fig. 4m–o ) and expected from equation (3). For RCP light, the opposite trend is observed ( Fig. 4g–i ). The measured m =+1 order’s power increases to ~76%, while the m =−1 order’s power approaches zero, again in agreement with simulations ( Fig. 4p–r ) and expected from equation (3). To further quantify the performance, we consider the polarization extinction ratio. We define this as the ratio of the power in the order directed to the left (right) to the power directed to the right (left) for LCP (RCP) illumination. A high extinction ratio of 50 is obtained. The extinction ratio depends on the incident angle (see Supplementary Table 1 and Note 7 ). We measure the transmitted power as being 45% of the input power. This compares well to the value of 47% predicted by simulations. Simulations also predict that, through removal of the residual a-Si layer, the transmission can be increased to 92% providing an opportunity to further improve the efficiency of the CDBS. The performance of the CDBS also depends on the input wavelength, as shown in Supplementary Fig. 6 and Note 8 . Figure 3: Fabricated device and measurement setup. ( a ) Top-view scanning electron micrograph (SEM) of a fabricated chirality-distinguishing beam-splitter (CDBS) device (a-Si nanofin grating). Dashed red rectangle indicates unit cell. Scale bar, 1 μm. ( b ) Side-view SEM of a CDBS device. Nanofins are slightly tapered in the minor axis, whereas tapering in the major axis is negligible. Aluminium mask is visible in this SEM, but removed before optical measurements. Scale bar, 1 μm. ( c ) Experimental setup consists of a fiber-coupled laser ( λ =974 nm) whose beam is collimated and passes through a linear polarizer (LP: maintained at 45°) and a quarter-wave-plate ( λ /4) to generate the desired input polarization. Angle between zero-th and first order is measured to be 19°. Full size image Figure 4: Comparison between measurements and simulations. Measured intensities of ( a ) −1 order ( b ) zero order and ( c ) +1 order for linearly polarized illumination. Measured intensities of ( d ) −1 order ( e ) zero order and ( f ) +1 order for left-circularly polarized (LCP) illumination. Measured intensities of ( g ) −1 order ( h ) zero order and ( i ) +1 order for right-circularly polarized (RCP) illumination. Corresponding simulations for linearly polarized ( j – l ), LCP ( m – o ) and RCP ( p – r ) illumination. Simulations are performed for nanofins with top widths of 55 nm, base widths of 70 nm, lengths of 285 nm and heights of 1,500 nm. These dimensions are chosen to match those found from scanning electron micrographs of a fabricated chirality-distinguishing beam-splitter device, but with base width modified. Full size image We demonstrate a CDBS with a large extinction ratio. Our study extends the applications of dielectric gratings by discriminating the handedness of light. In principle, the device can operate with minimal loss at wavelengths longer than that corresponding to the band gap of silicon. One particularly compelling application is that of polarization-resolving image sensors. Conventional image sensors achieve colour separations through the use of pixel arrays, where the unit cell comprises a set of red/green/blue filters. In an analogous manner, one could realize a polarization-resolving image sensor by employing polarization-splitting pixel arrays. In addition to a CDBS, each unit cell would contain elements to split linear polarizations. Such a device would present the opportunity for polarization-resolved imaging with very high efficiency, due to the fact that, based on their polarization, incoming photons would be redirected to the appropriate photodetector, rather than absorbed by a filter (as done in current approaches). In addition to pixel arrays, our method could enable the realization of more complex beam-shaping elements, achieved by other spatial modulation patterns of the nanofins in the x–y plane. The latter is under investigation. CDBS fabrication The starting substrate is a glass wafer that is cleaned using acetone (with sonication) followed by an oxygen plasma. Plasma-enhanced chemical vapour deposition is then used to deposit a-Si to a thickness of 1,680 nm. The a-Si deposition incorporates phosphorus doping to prevent problems related to the charging of the glass substrate that could otherwise occur during the electron beam lithography that is next. The wafer is spin coated with poly(methyl methacrylate) (PMMA, 495 K A2) at a speed of 6,000 r.p.m. and baked on a hotplate at 180 °C for 5 min. Next, the wafer is spin coated with PMMA (950 K A2) at a speed of 6,000 r.p.m. and baked on a hotplate at 180 °C for 5 min. This results in a PMMA bilayer. Electron beam lithography is then carried out (Elionix ELS-F125, 125 kV). The exposed resist is then developed in a mixture of methyl isobutyl ketone and isopropyl alcohol (MIBK:IPA is 1:3) at room temperature for 90 s, dipped in IPA for 30 s and blown dry using nitrogen. Aluminium (Al, 40 nm) is then deposited by electron beam evaporation at a rate of 2 Å s −1 . The lift-off process is then performed by soaking the sample overnight in a solvent stripper (Remover PG from Microchem). Inductively coupled plasma-reactive ion etching is then performed to etch the nanofins. The sample is then ashed in an oxygen plasma at 150 W for 5 min to remove the passivation layer generated during the etching process. The Al mask is removed by soaking in developer (MF319 from Shipley) for 5 min. The overall extent of the CDBS, that is, the nanofin grating, is 125 × 125 μm. To facilitate the optical characterization that occurs next, we add a metal layer to block the transmission of light through surrounding areas. This is done by performing optical lithography to define a resist square that coats the CDBS device, evaporation of titanium (5 nm, for adhesion) and nickel (145 nm) and the lift-off process. Measurements and simulations The measurement setup consists of a fiber-coupled laser ( λ =974 nm) whose beam is collimated by an objective lens ( × 10 magnification). The beam then passes through a linear polarizer and a quarter-wave-plate. In all measurements, the linear polarizer axis is maintained at 45°, while the quarter-wave-plate is adjusted to generate the desired linearly- or circularly polarized light. Light transmitted through the CDBS is either captured by a camera to record the beam profile or collected by a photodetector to measure the power. When used, the camera sensor is ~12 cm from the CDBS device. 3D simulations of the CDBS device are performed using the FDTD method (FDTD Solutions package from Lumerical Inc.). We apply periodic boundary conditions at the x - and y -boundaries and PMLs at the z -boundaries. The mesh spacing in the x - and y -directions is 5 nm, while it is 10 nm in the z -direction. The effective mode indices of the nanofins are calculated using 3D simulations (Mode Solver module, RSoft). Mesh sizes of 5, 1 and 5 nm are employed for the x -, y - and z axes, respectively. How to cite this article: Khorasaninejad, M. & Crozier, K. B. Silicon nanofin grating as a miniature chirality-distinguishing beam-splitter. Nat. Commun. 5:5386 doi: 10.1038/ncomms6386 (2014).